Parallel photonic information processing at gigabyte per second data rates using transient states The increasing demands on information processing require novel computational concepts and true parallelism. Nevertheless, hardware realizations of unconventional computing approaches never exceeded a marginal existence. While the application of optics in super-computing receives reawakened interest, new concepts, partly neuro-inspired, are being considered and developed. Here we experimentally demonstrate the potential of a simple photonic architecture to process information at unprecedented data rates, implementing a learning-based approach. A semiconductor laser subject to delayed self-feedback and optical data injection is employed to solve computationally hard tasks. We demonstrate simultaneous spoken digit and speaker recognition and chaotic time-series prediction at data rates beyond 1 Gbyte/s. We identify all digits with very low classification errors and perform chaotic time-series prediction with 10% error. Our approach bridges the areas of photonic information processing, cognitive and information science. The past century has seen an unprecedented increase in information processing abilities. However, certain tasks are not efficiently solved by standard computers. Unconventional computation schemes and the inclusion of photonic hardware could provide new opportunities [1] , [2] , [3] , [4] , [5] . Photonics might extend and complement the repertoire of techniques for certain information processing tasks, with far reaching consequences [3] . Realizing learning-based computation by utilizing the nonlinear transients of standard photonic components could lead to a paradigm shift in the field of optical computing, away from binary-logic based methods, towards machine learning-based approaches using off-the-shelf, fast and power efficient devices. In particular, semiconductor lasers exhibit nonlinear interaction between the laser field and semiconductor medium, resulting in complex behaviour when subjected to feedback, electrical modulation or optical injection [6] . They are off-the-shelf, high bandwidth, power efficient components, and form the backbone of modern fibre communication. In this article, we implement the computational concept of reservoir computing (RC) [4] in photonics, in particular realizing the reservoir and information injection all-optically. At the same time, we boost the bandwidth compared with previous approaches by more than two orders of magnitude. We achieve this by utilizing the analogue transient dynamics generated by a semiconductor laser coupled to a fibre-optic feedback loop. Following the RC concept, we generate nonlinear transient states in the context of previous input responses. Consequently, the system is capable of processing temporal sequences of information. Computational concept Our computational concept is schematically illustrated in Fig. 1a (ref. 7 ). Following ideas introduced in RC, we generate transient states for processing the information. These transient states are generated by a central nonlinear element, here a semiconductor laser, which is subjected to optical feedback with delay τ D , and to injection of the input information. The input information is sampled in time, resulting in a discrete sequence a n , n ={0,1,…}. In the case of real-time processing, the sampling rate should be chosen as T 2 −1 = τ D −1 . For successful information processing, a significant number of different nonlinear transients is required. In the case of a scalar input, we multiply a n by a temporal mask sequence M ( t ), the duration of which is equal to the sampling time T 2 . Each computational cycle T 2 is divided into N sub-intervals of duration T 1 = T 2 / N . With this procedure, we obtain N different, time-multiplexed transient states x m ( t ), with m =1… N and N typically chosen as 100≤ N ≤1,000. The resulting sequence injected into the laser during one delay time is therefore given by u n ( t )= a n · M ( t ). The induced nonlinear transient states have to contain a maximum amount of information about the injected input [7] . Therefore, we keep the system sufficiently far from reaching a steady state during its dynamical response. We achieve this by choosing T 1 =Θ· T 0 , with Θ=0.2, where T 0 is the characteristic time scale of the laser’s relaxation oscillations (ROs). In the case of multiple component input a n , the information injected each T 1 consists of a random, linear combination of input components. 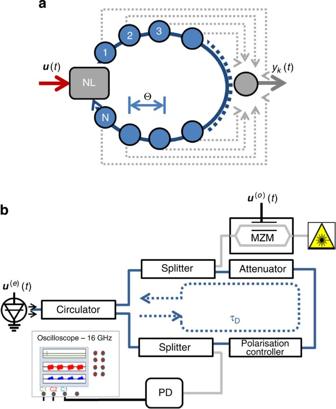Figure 1: Reservoir computing concept and experimental scheme. (a) Schematic representation of computation using nonlinear transient states generated by a single nonlinear element (NL) subject to delayed feedback. TheNtransient statesxm(t) used for computation are distributed along the delay line with spacing Θ. Here,ustands for the information input,yk(t) for the value of the readout with indexk. Panel (b) schematically shows the experimental realization of all-optical computation, utilizing a semiconductor laser diode as the nonlinear node. Information can be injected optically (electrically), given byu(o)(u(e)). The feedback delay is given byτD. The experimental setup comprises the laser diode, a tunable laser source to optically inject the information, a Mach–Zehnder modulator (MZM), a polarization controller, an attenuator, a circulator, splitters and a fast photo diode (PD) for signal detection. Figure 1: Reservoir computing concept and experimental scheme. ( a ) Schematic representation of computation using nonlinear transient states generated by a single nonlinear element (NL) subject to delayed feedback. The N transient states x m ( t ) used for computation are distributed along the delay line with spacing Θ. Here, u stands for the information input, y k ( t ) for the value of the readout with index k . Panel ( b ) schematically shows the experimental realization of all-optical computation, utilizing a semiconductor laser diode as the nonlinear node. Information can be injected optically (electrically), given by u (o) ( u (e) ). The feedback delay is given by τ D . The experimental setup comprises the laser diode, a tunable laser source to optically inject the information, a Mach–Zehnder modulator (MZM), a polarization controller, an attenuator, a circulator, splitters and a fast photo diode (PD) for signal detection. Full size image The final step in our computational process is based on the summation of these induced transient states x m ( t ). This is done by calculating a linear combination of the laser output intensities, detected at a rate of T 1 −1 . The coefficients of this linear combination, called weights, are determined by a standard machine learning training procedure, in which the difference between the resulting readout value and its target is minimized. Owing to the delay loop, the induced transients are the system’s response to the currently injected information in the context of the response to previous inputs. Theoretical [8] , [9] and experimental [7] , [10] , [11] , [12] investigations show that our scheme can indeed be interpreted as RC. For successful and reproducible computation, the system has to be capable of generating consistent transients, that is, for identical or highly alike inputs the induced transients have to be equally alike. This requirement corresponds to the approximation property in machine learning [4] , [7] . Therefore, the rest state (reservoir state in the absence of input) and the dynamical properties have to be chosen appropriately. Hence, computational performance benefits from a reservoir rest state corresponding to steady state emission of the laser. In the experiment, this can be achieved by, for example, biasing the laser close to the threshold current of the free running laser. Our scheme combines photonics with the true parallel computation properties of RC. First, the transients are induced by injecting information from multiple sources simultaneously into the laser. Second, as the transient states are not affected by the training, in principle, an arbitrary amount of k scalar outputs can be defined and trained, performing different computations. Parallel data injection can be realized using a single optical fibre without crosstalk between the individual input channels. Although, at this stage, data preprocessing and readout are carried out off-line, hardware implementations for a real-time preprocessing are being discussed [2] . Additional information about data injection and data readout can be found in the Methods section. Experimental scheme A schematic representation of the experimental setup is given in Fig. 1b . The emission of the semiconductor laser diode ( λ =1,542 nm) is collected by a standard single mode fibre. Feedback (with delay τ D =77.6 ns) is realized via a fibre loop, comprising an optical circulator, two fibre splitters, an optical attenuator and a polarization controller. The optical attenuator and polarization controller facilitate the control of the optical feedback conditions. Using T 2 =77.6 ns and N =388, we obtain T 1 =200 ps. In our experiment, information can either be injected electrically, via modulating the laser diode current, or optically by injecting the modulated intensity of a tunable laser. Diode current modulation was facilitated by directly connecting the diode to a radio frequency cable using a 40 Ω resistor. Combined with the 10 Ω impedance of the laser diode, the system therefore was impedance matched to the radio frequency electronics used for electrical modulation. Following this approach, we achieved a diode current modulation bandwidth exceeding 10 GHz. For electrical modulation, the laser’s RO frequency acts as bandwidth limiting factor. In our laser, the RO frequency changed from 1.4 to 5 GHz when changing the bias current from I b =9 mA to I b =20 mA. The optical signal was injected via the optical fibres forming the delayed feedback loop. In principle, efficient nonlinear interactions of optical signals in semiconductor lasers can be achieved for frequencies up to several hundreds of gigahertz [13] . So far, however, the signal source used for generating the input information remains the bandwidth limiting factor in our experiments. We evaluated the performance of our system focusing on two different, general classes of information processing tasks. Various information-processing problems require classification of information, associating different inputs to different classes. As such, these tasks equally require discrete classes as classifier targets, and a system response sufficiently diverse to allow for clear separation. A second typical task in information processing is based on nonlinear processing of dynamical information. Accordingly, the classifier target values can be continuous. Furthermore, the system has to provide memory to capture the dynamical nature of the injected information. We selected two computationally challenging tasks, each representing one of the two introduced classes of information processing tasks, as benchmark tests to evaluate the information processing capability of our scheme: parallel spoken digit/speaker recognition and chaotic time-series prediction. Both tasks are standard to the machine learning community and allow for a direct comparison between different approaches to information processing [7] , [10] , [11] , [14] . Spoken digit recognition In Fig. 2a we show the experimental results of spoken digit classification in terms of the classification error as a function of the laser bias current ( I b ). Results of optical (electrical) information injection are given by the blue (red) data set. Optical information was injected using a tunable laser, the polarization of which was parallel to the laser emission, with the optical injection power modulated between 15 nW ≤ u o ( t )≤15 μW. In the absence of information, that is, the rest state, the injected power corresponded to 15 nW. Electrical information was injected by modulating the laser current between 0 mA ≤ u e ( t )≤12 mA. The optical feedback was attenuated by 20 dB and rotated in polarization. Under these conditions, we achieved a very low classification error of (0.014+0.051/−0.014)% for I b =7.7 mA ((0.64±0.17)%, I b =7.6 mA) for optical (electrical) injection at a laser bias current close to the laser threshold. A classification error of 0.014% corresponds to one misclassification per ∼ 7,000 digits, with an uncertainty that was limited by the size of the database. Our results present an improvement in classification error by a factor of ∼ 3 and in speed by a factor 260 when compared with previous, optoelectronic implementations of this information processing scheme [10] , [11] . 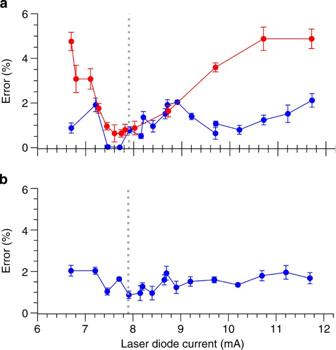Figure 2: Spoken digit classification with 5 GHz bandwidth. Blue (red) data correspond to optical (electrical) information injection. The same reservoir responses for identifying the digit (a) and the speaker (b) demonstrate the potential of RC for true parallel computation. Best performance is found for a laser diode currentIbclose to threshold (grey dotted line). A 20-fold cross-validation was repeated several times, with the s.d. given by the error bars. Figure 2: Spoken digit classification with 5 GHz bandwidth. Blue (red) data correspond to optical (electrical) information injection. The same reservoir responses for identifying the digit ( a ) and the speaker ( b ) demonstrate the potential of RC for true parallel computation. Best performance is found for a laser diode current I b close to threshold (grey dotted line). A 20-fold cross-validation was repeated several times, with the s.d. given by the error bars. Full size image We speculate that the improved error, as compared with earlier experiments [7] , [10] , [11] , [14] , is related to the influence of the nonlinearity on the classification performance. Such an influence has been empirically identified in Larger et al. [10] A thorough understanding of the interplay of nonlinearity and specific task performances is, however, still lacking. Even when compared with software emulations of neural networks, our performance is highly competitive. There, for the spoken digit recognition without the influence of noise, classification errors reported for a system based on hidden Markovian models were 0.168% (ref. 15 ), and 0.5% for a reservoir computing system [16] . Further above threshold, our system exhibits complex dynamics even in the absence of injected information [6] , yielding a worse performance for the case of electrical modulation ( Fig. 2a ). For the case of optical information injection the performance dependence above threshold is less intuitive. This might be due to the complex influence of the injected light on the stability of the rest state [17] . As an illustration of the parallel computation capabilities we utilized the same transient responses to identify the speaker of a digit. The results are shown in Fig. 2b . A (0.88±0.18)% speaker classification error was obtained for a bias current of I b =7.91 mA. At this point it is worth emphasizing the high speed of our setup, which allows us to process about one word in 3.3 μs, corresponding to ∼ 300,000 spoken digits per second. Our results represent the lowest spoken digit classification error as well as the highest speed reported in the literature. Chaotic time-series prediction The time-series prediction task requires a single point prediction of an experimentally obtained chaotic time series, which was also used in the Santa Fe competition [18] . The performance, using optical data injection, is depicted in Fig. 3 . For time-series prediction, the classifier target value is a nonlinear transformation of several, continuously distributed, previous data points, and therefore is (quasi-) continuous. Consequently, noise has a direct impact on the accuracy of the classifier. In order to reduce noise, the range of optical modulation was the same as before, however, an injection power of 7.5 μW was chosen, defining the rest state. The external laser therefore additionally served as an injection locking source, increasing the performance significantly by reducing the rest state noise. In our experiment, we performed a one-time step prediction test, that is, predicting a data-point one-time step ahead in the future. It is worth mentioning that we processed one data-point per delay time, and consequently no explicit memory was added at the data injection stage, a preprocessing technique commonly used to artificially introduce memory in machine learning techniques [19] . The quasi-continuous nature of our classifier is caused by the analogue-digital conversion in our experiment, which, in possible future applications, could be avoided. 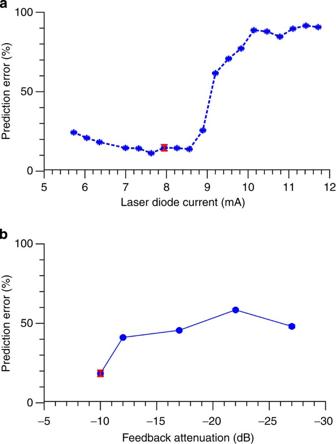Figure 3: Prediction error in a time-series prediction task. (a) Dependence on laser diode current using 10 dB feedback attenuation. (b) Dependence on feedback attenuation usingIb=7.9 mA. The prediction error increases dramatically forIb>8.9 mA, when the laser rest state becomes unstable. The importance of memory for time-series prediction can be seen in the lower panel, where the prediction error rapidly increases for a reduced feedback strength. Red error bars give the s.d. between three independent measurements. Blue error bars represent the s.d. for different training/testing partitions of the data. Figure 3: Prediction error in a time-series prediction task. ( a ) Dependence on laser diode current using 10 dB feedback attenuation. ( b ) Dependence on feedback attenuation using I b =7.9 mA. The prediction error increases dramatically for I b >8.9 mA, when the laser rest state becomes unstable. The importance of memory for time-series prediction can be seen in the lower panel, where the prediction error rapidly increases for a reduced feedback strength. Red error bars give the s.d. between three independent measurements. Blue error bars represent the s.d. for different training/testing partitions of the data. Full size image The prediction performance, depending on the bias current, is depicted in Fig. 3a . The best performance is again obtained for I b close to the laser threshold, with a prediction error of 10.6% ( I b =7.62 mA, feedback attenuation 10 dB) at a prediction rate of 1.3 × 10 7 points per second. When repeating the same input five times and averaging the responses (keeping the 8 bit resolution), the signal-to-noise ratio was improved, and an error of only 5.5% was obtained. The signal averaging was executed directly at the acquisition stage. Experimentally, this procedure could be implemented by running five systems in parallel or by making a trade-off between speed and performance. Time-series prediction using machine learning techniques and realized in software, achieved errors below 1% (refs 20,21) [20] , [21] . These approaches, however, neglect the influence of noise and finite experimental precision and, more importantly, add external memory in the data injection procedure. Although these implementations, for now, offer superior accuracy, hardware systems could offer advantages in speed, integrability and energy efficiency. These points will be discussed later in the manuscript. The importance of the memory introduced by the feedback loop can be seen in Fig. 3b . Owing to experimental constraints, the lowest feedback attenuation that we achieved was 10 dB, for which the best prediction performance was obtained. An increase by only 2 dB resulted in a prediction error exceeding 40%. We would like to emphasize that the data point with the lowest error in Fig. 3b does not stem from an individual measurement, but was confirmed by several independent measurements. The s.d. (±1.9%) of these measurements is given by the red error bars in Fig. 3 . Additional deviations arise from the cross-validation procedure. The entire training and testing procedure was carried out five times, using each data point for training and testing according to a random selection. Prediction results showed small deviations ( ∼ 0.3%) for different partitions. This error is displayed by the blue error bars in Fig. 3 . The direct influence of I b on the transient responses can be seen in Fig. 4 . Panel (a) shows a part of the Santa Fe time series used in the experiment, illustrating the sudden changes in amplitude, which are characteristic to this data set. Time-series prediction in the vicinity of these points is deemed particularly hard. Transients, induced by data containing such a rapid amplitude change, are displayed for three values of I b in panel (b). Although for I b =7.62 mA the dynamics is largely dominated by the system’s response to the injected information, this correlation between input and transient response reduces for larger I b . For a bias current of I b =10.78 mA, the characteristic amplitude change within the injected data is no longer vivid in the induced transients. The high quality of our time-series prediction is illustrated in Fig. 4c , where we compare the target (black) with the predicted (red) time series. The predicted time trace includes data points in the vicinity to a rapid amplitude transition. Here, top and bottom horizontal axes display the time step number in the original target trace, and the temporal duration of the actual experiment, respectively. 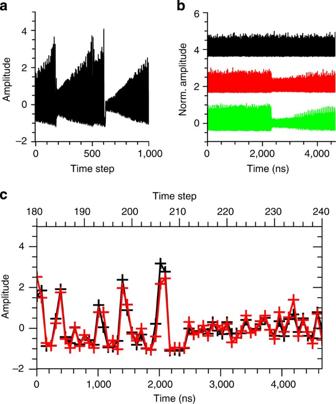Figure 4: Original and predicted trace and corresponding transients. A sample of the target time series can be seen in (a). Data displayed in (b,c) were obtained by injecting data from the 180th to 240th time step from panel (a). (b) Shows experimental transient states forIb=7.62, 9.2 and 10.78 mA, displayed in green, red and black, respectively. For high values ofIb, the transients lose the structure induced by the injected information, explaining the prediction error increase withIb. (c) Shows an example of the target (black) and predicted (red) time series forIb=7.6 mA. The top horizontal axis of panel (c) gives the times step number of the original target time trace, like given in (a). The lower horizontal axis represents the temporal duration for the prediction in the experiment, like given in (b). Figure 4: Original and predicted trace and corresponding transients. A sample of the target time series can be seen in ( a ). Data displayed in ( b , c ) were obtained by injecting data from the 180th to 240th time step from panel ( a ). ( b ) Shows experimental transient states for I b =7.62, 9.2 and 10.78 mA, displayed in green, red and black, respectively. For high values of I b , the transients lose the structure induced by the injected information, explaining the prediction error increase with I b . ( c ) Shows an example of the target (black) and predicted (red) time series for I b =7.6 mA. The top horizontal axis of panel ( c ) gives the times step number of the original target time trace, like given in ( a ). The lower horizontal axis represents the temporal duration for the prediction in the experiment, like given in ( b ). Full size image Apart from the demonstrated highly competitive figures of merit, our novel computational concept might offer significant energy reduction for certain tasks. At this stage we can only provide a conservative estimate. The calculated energy consumption for spoken digit recognition using our all-optical transient computing scheme, including all-optical data input and readout hardware, would be of the order of 10 mJ per digit, compared with 2 J per digit required by a standard desktop computer. These numbers demonstrate the great potential of our computational scheme realized in hardware. Additional information about the energy consumption can be found in the Methods sections. Other hardware implementations of machine learning concepts are based on field programmable gate arrays. There, the states utilized for computation are realized based on digital electronics. The speed of these implementations is measured in connections per second, with the fastest systems typically achieving rates from 1 × 10 9 to 5 × 10 9 connections per second for a single field programmable gate arrays [22] . It is worth noting that this number refers to connections and not to the number of nodes of the neural network, hence a more complex network structure will inevitably decrease the global processing rates. Our scheme, with the injection rate limited by our signal source, therefore allows for identical or even superior processing speed. In conclusion, we have experimentally demonstrated the computational power of a single photonic device using nonlinear transient laser responses. The reported results open new perspectives for tackling certain tasks with analogue optical computation. Instead of relying on complicated, power- and space-consuming architectures, one can realize simple, yet powerful implementations of optical information processing with inherent memory and the possibility of true parallelism. Of major consequence might be the large computational power achieved with the nonlinearity of a laser diode. Similar computational schemes could in the future be implemented, benefiting from the vast variety of optical nonlinearities already available. As such, implementations could span numerous areas, including ultra-fast optical nonlinearities, some even on the femtosecond time scales, as well as utilizing nano-and metamaterials. We achieved excellent figures of merit in spoken digit recognition, with the lowest reported error rate (0.014%) at simultaneously highest data rate (1.1 Gbyte/s), and time-series prediction with an error of only 10.6% with a prediction rate of 1.3 × 10 7 data points per second. Especially for optical information injection, the factor ultimately limiting the speed of this scheme might not arise from the maximum bandwidth of the photonic nonlinear element [13] , but from a decreasing signal-to-noise ratio when going to higher bandwidths. Using a slightly modified injection scheme, demonstrated in the time-series prediction task, we have shown how these effects can, to some degree, be compensated for. We would like to point out that for all tasks, digit and speaker recognition as well as time-series prediction, best performance was achieved for laser bias currents close to threshold. Consequently, the main parameter determining the performance does not require a fine adjustment for executing different tasks. For tasks requiring extended or multiple time scale memory, our scheme can be expanded by utilizing several delay lines of different length [14] or by adding additional nonlinear nodes (lasers). Our results, reported for the two different tasks, indicate the potential of our information processing schemes and open new perspectives for future applications in photonics. Spoken digit recognition is a classification task, and as such our excellent figures of merit might be transferable to technological challenges like all-optical routing [23] . However, tackling all-optical routing with the implementation as presented would currently still be out of reach becaus of the employed time multiplexing. A possible extension includes the use of a multiple node reservoir, based on semiconductor lasers. With such extended schemes, data rates of tens of gigabit per second should be achievable. Furthermore, based on the all-optical nonlinearity of laser diodes [13] , such systems might even reach processing speeds of hundreds of gigahertz. These numbers demonstrate the potential of RC based on off-the-shelf photonic components for telecommunication applications. However, many questions still need to be investigated on the way. The fast speed and good performance in time-series prediction equally demonstrate possible applications in ultra-fast control system. Here, the increase to tens of megahertz bandwidth could offer great opportunities for fast control of photonic systems. In addition, the simplicity of our scheme could allow technological implementations in distributed networks and smart systems, enabling closed loop control of individual elements. Information injection and readout In our experiment, the information to be processed can be injected either electrically, via directly modulating the laser bias current ( u ( t ) (e) ), or optically via modulating the optical intensity of an external injection laser using a Mach–Zehnder modulator ( u ( t ) (o) ). In both cases, the modulation rate is given by T 1 −1 =(Θ· T 0 ) −1 . We chose Θ such that a high sensitivity of the induced transient states on the injected information is achieved, which we find optimized for Θ ∼ 0.2. Larger Θ values would allow the induced transient to approach their steady state, while for too small Θ values the system’s inertia would result in a neglegible response to the injected information. Input information for the n th input interval is described by the L -dimensional data vector a n . The data vector is created via sampling the input information in discrete time steps. For realizing parallel injection of the L- dimensional input, we construct vector ũ with N dimensions according to where is a connectivity matrix, defining connections between input dimensions and the individual transients. A large diversity of transient states is required in our computational scheme. This is achieved by an additional multiplication of vector ũ with mask M ( t ). According to this, mask M defines the temporal position m · T 1 of vector components u n , m inside one clock cycle T 2 . The mask is defined as a sequence of N values, randomly selected from discrete values. For the temporal interval, defined by ([ n · T 2 +( m −1)· T 1 ]≤ t <[ n · T 2 + m · T 1 ]), the information injected into the reservoir is given by The resulting, u ( t ) is the information directly injected into the nonlinear node. Following these data injection procedure, it is possible to inject L data values in parallel into the nonlinearity during one computational time step T 2 . For the training, standard methods from machine learning can be employed [4] . In our computational scheme, the processed information is represented by scalar values y k of the individual classifiers, indicated by k . Combined, these values (dimensions) form the output vector y . Per time step T 2 one computation is executed, hence we normalize time according to s = t / T 2 . The output vector is given by where the matrices contain a linear combination of the transient states, generated by the information injected into the laser and a constant bias term, respectively. For performing a certain information processing operation on readout vector y , the linear weights are determined in a training procedure. Information with known target values is injected into the system to optimize . Consequently, the s.d. between y ( s ) and its target is minimized. During this procedure, referred to as training, the readout weights are adjusted in an off-line procedure. For the case of an input with s time steps, we build a transient state matrix of dimension N × s , containing all transient states at each time s . To account for a constant offset in the target value, we additionally include a constant bias, resulting in a state matrix of dimension ( N +1) × s . Furthermore, we concatenate all readout weights defining matrix . For a number of k individual readouts y , the dimensionality of is k × ( N +1). We define a target output matrix , given the optimal output values at each time step (that is, dimension k × s ). Using these three matrices, the root mean square can be minimized according to Here, † denotes the Moore–Penrose pseudo-inverse, which allows to avoid problems with ill-conditioned matrices. Over-fitting of the training data is avoided by the noise inherently present in the experiment, and by the Tikhonov regularization method (ridge regression). Tikhonov regularization is included in the training procedure by minimizing where the factor λ acts as a penalizing factor, forcing the components of towards smaller values. Spoken digit recognition The spoken digit data set consists of five female speakers, uttering the numbers zero to nine with a tenfold repetition for statistics [24] . Before injecting the information into the laser, we performed standard preprocessing creating a cochleagram of each digit via the Lyon ear model [25] . For simplicity, mask M and connectivity matrix were merged into a single matrix . In this matrix, 98% of the elements were set to zero in order to realize a sparse connectivity between cochleagram channels and transients. The remaining values were randomly selected among (0.41,0.59). The preprocessing following the digit’s chocleagram is illustrated in Fig. 5 . After preprocessing, each cycle of length T 2 data of the cochleagram’s 86 frequency channels were injected into the system with 8 bit resolution, corresponding to a rate of 1.1 Gbyte/s. One Byte here refers a unit of injected information, which can comprise different numbers of bits. Out of the entire body of spoken digits, we chose 20 random partitions of 25 samples each, using 475 samples for training the readout weights, keeping the remaining 25 for testing. Each random partition and each sample are used exactly once for testing (20-fold cross-validation). Statistical information is provided by repeating this procedure five times, creating different random combinations of testing and training. At the two data points, where the system approaches 0% error, the cross-validation procedure was repeated 100 times. 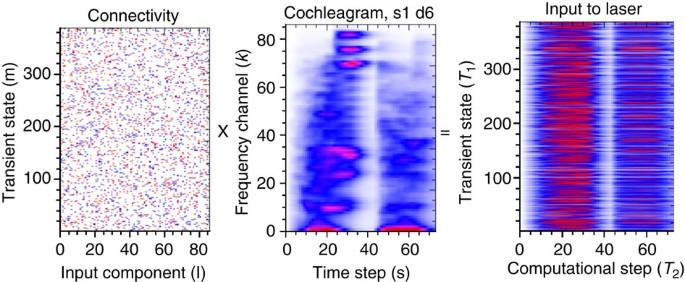Figure 5: Matrix multiplication to generate input to laser. Cochleagram of digit six, uttered by speaker one is multiplied by matrix, creating the laser input. Figure 5: Matrix multiplication to generate input to laser. Cochleagram of digit six, uttered by speaker one is multiplied by matrix , creating the laser input. Full size image Time-series prediction In the time-series prediction task the system was injected with one data point per T 2 . The target of the classifier was to predict the value of the respective next time step. By injecting information at a rate of 1 Byte per clock cycle T 2 (1 Byte=8 bits), we could predict 1.3 × 10 7 data points per second. We evaluated the performance of our scheme using the chaotic time-series of the Santa Fe time-series competition, data set A (ref. 18 ). The data set, created by a far-infrared-laser operating in a chaotic state [26] , consists of 4,000 data points, from which we used 80% for training and 20% for testing and five-fold cross-validation. The input information for the time-series prediction task consisted of scalar values only. Accordingly, input and transient states are fully connected. Time-series prediction is very sensitive to the presence of noise. To evaluate the performance of our system, we carried out numerical simulations, that showed that for an 8-bit digital to analogue converter digitization noise would already limit the performance of our system. A mask with a larger variety of values can reduce the performance limiting influence of this factor to some extent [27] . Hence, for this task we employed a six-valued mask, with a random selection from the values {−1, −0.6, −0.2, 0.2, 0.6, 1}. An additional positive effect of this injection scheme is that a single value of the injected information is the origin of all N transient states during one delay. The impact of noise is therefore reduced by averaging over the large number of states, hence increasing prediction accuracy and robustness. It is worth noting that in our experiments we aim at demonstrating time-series prediction utilizing only the memory inherently present in the system. For this reason, we inject a single data point per delay T 2 . Injecting multiple points within one delay time would result in an artificial enlargement of the memory. Energy efficiency estimation The energy consumption for a system, entirely realized in hardware, was calculated using off-the-shelf components. Masking of the input and realizing the scalar multiplication factors in the readout classifier can, due to the time multiplexing, be done via temporal amplitude modulation (for example, with a Mach–Zehnder modulator). The readout additionally requires integration for the duration of T 2 . This can be realized electronically with a gated integrator [28] or optically with an all-optical integrator [29] . Our calculations are based on the gated integrator, for which we estimate a power consumption of 200 mW. The temporal modulation sequence for the input and readout is provided by an arbitrary waveform generator (AWG, Euvis AWG452), with a power consumption of 13 W. One AWG for each input and output were used in our estimation which gives an upper limit for the power consumption, with large potential for further reductions. We assumed the transformation by the Cochleagram to be carried out in advance. As such, a system with 10 classifiers would consume roughly ∼ 150 W. We included an additional 50 W for all other components like the laser diode current source and temperature stabilizer, as well as the driver of the Mach–Zehnder modulator. This number does not rely on any specifically designed electronic hardware, and hence represents a highly conservative guess. How to cite this article: Brunner, D. et al. Parallel photonic information processing at gigabyte per second data rates using transient states. Nat. Commun. 4:1364 doi: 10.1038/ncomms2368 (2013).